Diversity of trion states and substrate effects in the optical properties of an MoS2monolayer Almost all experiments and future applications of transition metal dichalcogenide monolayers rely on a substrate for mechanical stability, which can significantly modify the optical spectra of the monolayer. Doping from the substrate might lead to the domination of the spectra by trions. Here we show by ab initio many-body theory that the negative trion (A − ) splits into three excitations, with both inter- and intra-valley character, while the positive counterpart (A + ) consists of only one inter-valley excitation. Furthermore, the substrate enhances the screening, which renormalizes both band gap and exciton as well as the trion-binding energies. We verify that these two effects do not perfectly cancel each other, but lead to red-shifts of the excitation energies for three different substrates ranging from a wide-bandgap semiconductor up to a metal. Our results explain recently found experimental splittings of the lowest trion line as well as excitation red-shifts on substrates. Semiconducting transition metal dichalcogenides (TMDCs) have attracted much attention as candidates for future opto-electronic applications due to their particularly rich physical properties: the indirect-to-direct band-gap transition from bulk to monolayer [1] , [2] , selective valley- and spin-excitations [3] , [4] , [5] , [6] , [7] , and high on–off ratios as field-effect transistors [8] . Because of their two-dimensional nature, most of the measurements of these properties demand a substrate supporting the monolayer. The combination of the two-dimensional structure and enhanced Coulomb interaction causes strong excitonic effects in the monolayers, with reported binding energies of several hundred meV in MoS 2 [9] , [10] , [11] . In addition to excitons, Coulomb interaction can cause the preferred formation of trions, which often dominate the photoluminescence spectra when free charges are present [12] , [13] , [14] , [15] , [16] , [17] , [18] , [19] . These additional charges can stem from gating, defects, or from a substrate that is used for mechanical stability, a process frequently reported in mechanically exfoliated MoS 2 monolayers [20] , [21] . Depending on the type of the additional charges (electrons or holes) either negative or positive trions will form. While trions have been discussed for quantum dots and similar structures, only few theoretical studies have looked into their properties for TMDCs so far. Experimentally, Ross et al. [13] used an externally applied voltage that allowed to control the charge of the excitation moving from negative trions to neutral excitons, and further to positive trions. Further studies reveal a splitting of the trion line [22] , as well as asymmetric photoluminescence intensities [22] , [23] . In addition, those trions corresponding to the second lowest exciton (B) have been observed [24] . These experimental findings underline the need for a theoretical approach that yields both the complete exciton and trion spectra. The goal of this work is to address these experimental findings, i.e., to understand the interplay between a TMDC monolayer and a substrate, including the formation and properties of both negative and positive trions and the role of the additional substrate screening quantitatively [25] . For this we apply the framework of ab initio many-body perturbation theory (MBPT, see Supplementary Notes 1 and 2 ) [26] , [27] and extend it to include trions (Supplementary Note 3 ). Our computational first-principles approach allows a detailed look into the trion spectra and wave functions in real and reciprocal space, revealing the energetically lowest trion (A − ) as split into three excitations with both inter- and intra-valley character. Remarkably, the positive trion (A + ) behaves much different with only one energetically low-lying trion peak. Furthermore, the substrate necessarily contributes dielectric polarizability, and thus weakens the Coulomb interaction inside the TMDC monolayer [28] , [29] , causing spectral shifts of both exciton and trion energies as compared to the vacuum environment. It was demonstrated in several works that the screening enhancement causes both strong band-gap renormalization and a reduction of the exciton-binding energy [29] , [30] , [31] , [32] . Here we extend the previous findings and verify that these two large effects do not exactly cancel each other, instead they result in small, but robust shifts of both the excitonic and trionic transition energies to the red (lower energies) for TMDC monolayers. Trion excitations TMDC monolayers often exhibit a second kind of excited state next to excitons: trions [12] , [13] , [14] , [15] , [16] , [17] , [18] , [19] . They result from the correlation between three excited particles, either two electrons and one hole or one electron and two holes, depending on the type of doping. These additional charges can, for example, be provided by the substrate [20] , [21] . Experimentally, their transitions are commonly found at energies slightly below those of excitons. Theoretically, parameter-based descriptions through a model Hamiltonian [33] , [34] , [35] , [36] , [37] form an established approach toward these three-particle excitations, predicting binding energies of the A − trion in MoS 2 of 26–32 meV [38] , [39] . Going beyond these approaches, we extend the concepts of MBPT resulting in an ab initio method [40] that is generally applicable to all systems, overcoming system-specific modeling. We include the full band structure (instead of an effective mass approach) with interband mixing, and as output get the complete trion spectrum, including dark states, and the full atomically resolved trion wave functions in real and k -space (for details of the method and numerical convergence see “Methods” section, Supplementary Figs. 1 – 6 and Supplementary Notes 1 – 6 ). Our approach is implemented for both negative and positive trions. Furthermore, we are able to quantify the effect of the substrate screening on trions. 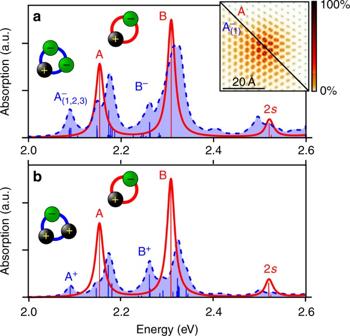Fig. 1 Exciton and trion spectrum of an MoS2monolayer. The excitonic contribution to the optical absorption spectrum is shown in red. The trionic contribution (shown in blue, referring to negative trions inaand positive trions inb) exhibits resonant states (close to the A and B exciton) and bound states (red-shifted compared to the corresponding excitons). The A−trion is split into three separate peaks, labeled\({\mathrm{A}}_{(1,2,3)}^ -\). The numerical recursion scheme64is used to calculate the energetically lowest states. For the spectra above 2.3 eV inaand 2.4 eV inb, the Haydock recursion scheme is applied. An artificial broadening of 0.01 eV is used. Inset: comparison between the real space electron distribution (in arbitraty units) of the A exciton with the electron distribution from the\({\mathrm{A}}_{(1)}^ -\)trion (see Supplementary Fig.7for details). For this, the hole is fixed in the center of the panel close to a Mo atom, in which the distribution is shown. For the trion state, the distribution of one electron is shown after complete spacial averaging over the second electron Figure 1 shows both the absorption spectrum derived from first principles due to excitons in red (showing the prominent A and B excitons as well as the A 2 s exciton) and due to trions in blue for a MoS 2 monolayer as a representative for the whole class of TMDCs. We note that the A 2 s exciton is not completely converged (Supplementary Fig. 4 ). The first point that is striking in both trion spectra (negative trions in a and positive trions in b) is the huge variety of excitations compared to only two excitons below 2.4 eV. Resonant trions are found close to the A and B excitons, accompanied by bound trions that lie red-shifted below the excitons (A − , A + and B − , B + ). Interestingly, the A − trion is split by 1 and 4 meV into three separate peaks, \({\mathrm{A}}_{(1,2,3)}^ -\) (for its detailed analysis see below). The trion-binding energy (in vacuum) is found to be 43 meV for \({\mathrm{A}}_{(1)}^ -\) and 23 meV for B − as well as slightly lower for A + (39 meV) and B + (23 meV). Comparing the absorption intensities, we find that the negative A − trion absorbs more light than the positive A + trion. This is a direct consequence of the three peaks that form A − compared to only one in A + . We note that both results, the lower trion-binding energy of A + and the lower intensity are observed experimentally by Jones et al. [22] for WSe 2 , for which we expect similar results as for MoS 2 . Note that while we are able to compare the intensity of the trions relative to each other, the ratio between trion intensity and exciton intensity depends on the doping. As this is not explicitly taken into account in our calculation, we are not able to directly compare trion to exciton intensities in the spectra. Fig. 1 Exciton and trion spectrum of an MoS 2 monolayer. The excitonic contribution to the optical absorption spectrum is shown in red. The trionic contribution (shown in blue, referring to negative trions in a and positive trions in b ) exhibits resonant states (close to the A and B exciton) and bound states (red-shifted compared to the corresponding excitons). The A − trion is split into three separate peaks, labeled \({\mathrm{A}}_{(1,2,3)}^ -\) . The numerical recursion scheme [64] is used to calculate the energetically lowest states. For the spectra above 2.3 eV in a and 2.4 eV in b , the Haydock recursion scheme is applied. An artificial broadening of 0.01 eV is used. Inset: comparison between the real space electron distribution (in arbitraty units) of the A exciton with the electron distribution from the \({\mathrm{A}}_{(1)}^ -\) trion (see Supplementary Fig. 7 for details). For this, the hole is fixed in the center of the panel close to a Mo atom, in which the distribution is shown. For the trion state, the distribution of one electron is shown after complete spacial averaging over the second electron Full size image Trion wave function and band composition The modulus squared of the real space wave function of the first bright negative-trion peak \({\mathrm{A}}_1^ -\) is plotted in the inset of Fig. 1a along with the respective distribution for the A exciton. For both, the hole is fixed at the same position close to a Mo atom, and one electron of the trion is spatially integrated out. The result is an insight into the real-space distribution of the trion state, which is much widely extended than the corresponding exciton. We find the root-mean-square radius of the exciton distribution to be \(\sqrt {\left\langle {{\mathbf{r}}^2} \right\rangle } = 8.8\) Å, while the corresponding value of the trion distribution is ~30% larger at 11.4 Å. This is a direct consequence of the additional repulsive force between the two electrons involved in the trion state. For a deeper understanding of the \({\mathrm{A}}_{(1,2,3)}^ -\) trions, we investigate their contributions in reciprocal space. 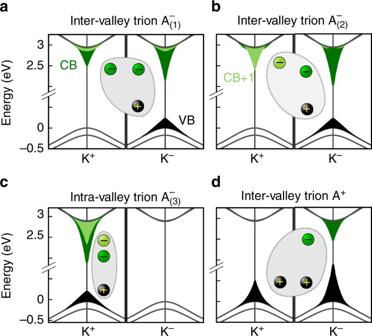Fig. 2 Quasiparticle band structure of an MoS2monolayer. The figure focuses on the vicinity of the K+and K−points.a–cFor all three negative trion excitations\({\mathrm{A}}_{(1,2,3)}^ -\)the band-resolvedk-dependent contributions (square of the wave functions) are attached to the respective bands (black for the VB and dark (light) green for the CB (CB+1)). For the\({\mathrm{A}}_{(1,2)}^ -\)trions the electrons are located in different valleys, while for\({\mathrm{A}}_{(3)}^ -\)only one valley contributes. The initial one-electron state resides at K+in the CB.dContribution of the A+trion, the initial hole resides at K+. We note that in addition to these trions with total momentum K+the same set of trions with exchanged K+↔ K−occurs forK= K− Figure 2 shows the quasiparticle band structure of the MoS 2 monolayer in vacuum around K + and K − , including the two highest valence bands (VBs) (spin-split by 175 meV) and the two lowest conduction bands (spin-split by 15 meV). Indicated in the band structure are the contributions of each band to all three \({\mathrm{A}}_{(1,2,3)}^ -\) trions (Fig. 2a–c ). These three lowest trions are all build up from the highest VB, and the two lowest conduction bands (CB, CB+1), but are still strikingly different. In the simplified picture of an electron bound to an exciton, the occurrence of three states can be easily understood. As the CB at the K valley is occupied by the electron of the bright exciton, the second electron can only reside in one of the other bands/valleys (Pauli exclusion). In addition to the three states shown here with a trion momentum of K = K + , the same set of excitations exist with K = K − (all contributions are found at the different valley K + ↔ K − ) summing up to six trions in total. While \({\mathrm{A}}_{(1,2)}^ -\) are located both at K + and K − (inter-valley), \({\mathrm{A}}_{(3)}^ -\) is exclusively located at K + (intra-valley). \({\mathrm{A}}_1^ -\) and \({\mathrm{A}}_2^ -\) can be distinguished by their spin character. While all electron spins point into the same direction for \({\mathrm{A}}_2^ -\) , the “additional” electron obtains a reversed spin in \({\mathrm{A}}_1^ -\) . The inter-valley trion \({\mathrm{A}}_1^ -\) is the energetically lowest conduction band. This can be understood since splitting the two electrons into two valleys allows them to both reside in the energetically lowest conduction band. Fig. 2 Quasiparticle band structure of an MoS 2 monolayer. The figure focuses on the vicinity of the K + and K − points. a – c For all three negative trion excitations \({\mathrm{A}}_{(1,2,3)}^ -\) the band-resolved k -dependent contributions (square of the wave functions) are attached to the respective bands (black for the VB and dark (light) green for the CB (CB+1)). For the \({\mathrm{A}}_{(1,2)}^ -\) trions the electrons are located in different valleys, while for \({\mathrm{A}}_{(3)}^ -\) only one valley contributes. The initial one-electron state resides at K + in the CB. d Contribution of the A + trion, the initial hole resides at K + . 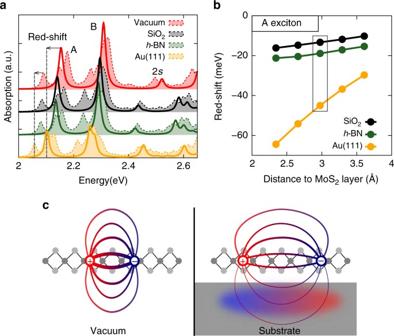Fig.3 Red-shift of optical transitions due to substrate screening.aExciton (solid lines) and negative trion (dashed and filled lines) absorption spectra of an MoS2monolayer in vacuum and on different substrates. Both spectra stem from a single calculation. The arrows indicate the red-shift in going from MoS2in vacuum to a gold substrate. All substrates are placed at a distance of 3 Å and have a well-converged thickness of about 10 Å (i.e., increasing the substrate thickness by another layer of ~2 Å leads to an excitation shift of less than 0.5 meV). An artificial broadening of 0.01 eV is used.bRed-shift of the A exciton energy as a function of the distance to the substrate (using extrapolated values ofN→ ∞ in thek-mesh). The box marks the distance used ina.cSchematically illustration of a bound electron–hole pair in vacuum and on a substrate, where the Coulomb interaction is screened and the substrate is polarized 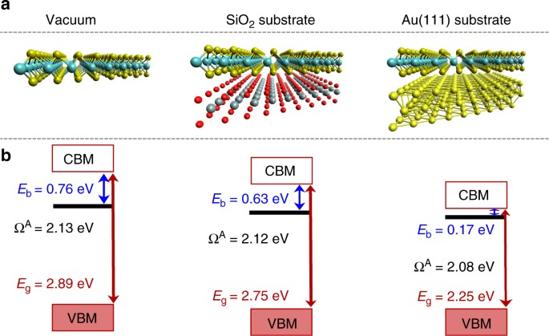Fig. 4 Energy composition of the A exciton on various substrates. We consider vacuum, an SiO2and an Au(111) substrate at a distance of 3 Å (seea). For each system the bandgapEg, the excitation energy ΩAand the binding energyEbare given inb We note that in addition to these trions with total momentum K + the same set of trions with exchanged K + ↔ K − occurs for K = K − Full size image Having discussed the splitting for MoS 2 , we note that it is quantitatively different in TMDCs, which include tungsten. Due to the interchanged character of CB and CB+1, we find that for WSe 2 , \({\mathrm{A}}_2^ -\) is moved 30 meV below \({\mathrm{A}}_1^ -\) and now constitutes the lowest trion state. Experimental confirmation of two different kind of trions and practical usability was shown in recent measurements on WSe 2 by Jones et al. [41] and on WS 2 by Boulesbaa et al. [42] . Yu et al. [43] offered a qualitative explanation for the different trions. Figure 2d shows the corresponding contributions to the A + trion. The lowest optical active state has inter-valley character, where both holes reside in the topmost VB and the electron in the CB at K − . The positive trions with one hole residing in the lower VB are not found in the vicinity of the A − trion due to the larger spin–orbit splitting in the VBs compared to the CBs. By considering all possible trion momenta, we find two low-energy states among the positive trions, while six low-energy states are observed among the negative trions. Further trions (positive and negative) are found at higher energy states. Finally, we note that the (negative) trion states can be distinguished by combining a spin-polarized doping (e.g., from a magnetized substrate) and the usage of circular polarized light. We expect \({\mathrm{A}}_1^ -\) and \({\mathrm{A}}_3^ -\) (with momentum K ) to be found with one light polarization, while \({\mathrm{A}}_2^ -\) (momentum − K ) may show up with light of the other polarization. If spin-polarized hole current is used to build up positively charged trions A + , we expect them to be only visible with one light polarization while the other will be dark. Effects of substrate screening A substrate might not only donate additional charges, but also drastically enhance the screening environment, which can be captured within our approach. The key results are summarized in Fig. 3a, which compares both the exciton and the negative trion spectra for vacuum, an SiO 2 , a h -BN, and a gold substrate. Compared to the free-standing monolayer in vacuum, both the excitons and the trions are red-shifted toward lower energy. Since negative doping through a substrate is frequently reported in TMDCs, we concentrate on negative trions for the substrate effects. The red-shifts of excitons and trions show two clear features: (i) They increase with the substrate polarizability, e.g., in the sequence vacuum → SiO 2 → h -BN → Au in our study (as illustrated by their dielectric constants of ε ∞ = 3.9 (SiO 2 [44] ), 4.95/4.10 ( \(\varepsilon _\infty ^{||}\) / \(\varepsilon _\infty ^ \bot\) h -BN [45] ), and ∞ (Au)). (ii) The red-shift increases with decreasing distance between substrate and monolayer. This trend can be seen in Fig. 3b for the A exciton. The smaller the distance, the stronger the screening which leads to a larger red-shift. At the typical van der Waals distance of ~3 Å, we observe red-shifts for the A exciton of 13 meV on SiO 2 , 19 meV on h -BN, and 45 meV on Au(111). Note that due to the involved approximations, the relative accuracy (as difference between two values) of our calculations is better than the absolute accuracy. Thus, red-shifts and trion-binding energies are given in meV (see also Table 1 ). Notably, the excitons experience a stronger shift than the trions, leading to a substrate-dependent trion-binding energy. Fig.3 Red-shift of optical transitions due to substrate screening. a Exciton (solid lines) and negative trion (dashed and filled lines) absorption spectra of an MoS 2 monolayer in vacuum and on different substrates. Both spectra stem from a single calculation. The arrows indicate the red-shift in going from MoS 2 in vacuum to a gold substrate. All substrates are placed at a distance of 3 Å and have a well-converged thickness of about 10 Å (i.e., increasing the substrate thickness by another layer of ~2 Å leads to an excitation shift of less than 0.5 meV). An artificial broadening of 0.01 eV is used. b Red-shift of the A exciton energy as a function of the distance to the substrate (using extrapolated values of N → ∞ in the k -mesh). The box marks the distance used in a . c Schematically illustration of a bound electron–hole pair in vacuum and on a substrate, where the Coulomb interaction is screened and the substrate is polarized Full size image Table 1 Energy composition of the A exciton and trions Full size table The usage of the atom-resolved model function of the LDA+GdW approach [46] allows a straightforward handling of the screening due to a substrate by including substrate atoms in the dielectric function (Supplementary Note 1 ). The used method was already successfully employed to describe excitons in WSe 2 monolayers [47] , and to include the screening of substrates for molecular adsorbates [48] , [49] . Note that in this approach the atoms from the substrate change the screening, but do not interact via chemical bonding with the monolayer. The role of screening has already been investigated in parameter-based [39] and parameter-free [29] , [50] approaches. Comparing vacuum and an SiO 2 substrate, Kylanpaa et al. have found a difference of 0.18 eV in exciton binding while we found 0.13 eV (Fig. 4 ). Due to the different inclusion of the substrate (homogenous vs. atomically structured) such a small quantitative difference is not astonishing. We underline that ref. [39] does not consider the concomitant change of the band-structure energies. Thus, they do not obtain the combined red-shift. Furthermore, some models might not be directly applicable to cases of metallic screening [39] . Fig. 4 Energy composition of the A exciton on various substrates. We consider vacuum, an SiO 2 and an Au(111) substrate at a distance of 3 Å (see a ). For each system the bandgap E g , the excitation energy Ω A and the binding energy E b are given in b Full size image There are a couple of experimental observations on exciton red-shifts in MoS 2 monolayers. Scheuschner et al. [19] measured the A − trion in a free-standing monolayer, as well as, on an SiO 2 substrate. The two data sets of Figure 8 of ref. [19] seem to indicate a red shift of about 25 meV. In a recent work by Klein et al. [51] an MoS 2 monolayer on a flat surface was subsequently covered by Al 2 O 3 . Comparison of the A exciton without and with the cover shows a red-shift of about 15 meV due to the Al 2 O 3 cover. In a further experiment, Lippert et al. [52] found a red-shift of the A exciton of a WSe 2 monolayer of 12 meV in changing substrates from SiO 2 to the stronger screening of a sapphire substrate. Red-shift of optical excitations To understand the spectral shifts in the absorption spectra (Fig. 3 ) we first focus on the excitons. Our calculations allow to identify the exciton red-shifts as a combination of two effects, which are summarized in Fig. 4a, b . First, the substrate renormalizes the fundamental bandgap of the MoS 2 monolayer. Starting from E g = 2.89 eV in vacuum, e.g., an Au(111) substrate reduce the gap by 0.64 to 2.25 eV. Bruix et al. [53] found a similarly small gap of 1.95 eV for MoS 2 on Au(111), clearly demonstrating the drastic band-gap renormalization (see also refs. [29] , [54] , [55] ). The physical origin of the reduction of the bandgap is the image charge effect [50] , [56] . The energy needed to introduce an additional electron into the system defines the conduction band minimum (CBM). If a substrate is present, the additional electron will contribute to its polarization, and thus reduce the total energy, shifting the CBM down. The opposite effect holds for the valence band maximum (VBM), thus closing the fundamental gap. Secondly, the exciton binding energy E b is reduced: Additional polarizability in the substrate reduces the Coulomb interaction between electron and hole (schematically depicted in Fig. 3c ). In the extreme case of the metallic substrate Au(111), the resulting exciton binding energy is 0.17 eV, which is only one-fifth of the vacuum value (0.76 eV). The reduced binding energy is directly visible in the exciton wave functions that gets more extended in real space. We find \(\sqrt {\left\langle {{\bf{r}}^2} \right\rangle } = (8.8{\mathrm{/}}9.5{\mathrm{/}}11.2)\) Å for vacuum/SiO 2 /Au(111), respectively (Supplementary Fig. 7 ). As a result of our study, we verified that these two large effects (the reduced binding energy and the closing of the gap) do not perfectly cancel each other, but lead to shifts in the excitation energies always to the red (lower energy) for physisorbed systems. Note that we expect that the physisorbed system does not change its structure or occupation when a substrate is introduced. Furthermore, it should not have a long-range static dipole (quadrupole, etc.) moment. A straightforward way of understanding why excitations always shift to the red is to imagine the excited state (and the corresponding total energy) with and without the substrate. The additional degree of freedom due to the surface polarizability will always lower the total energy. Furthermore, the substrate will adjust its charge density, known for metals as image charges [50] . This gained energy leads to a reduced excitation energy, i.e., a red-shift compared to vacuum. Such red-shifts have been reported in many materials [57] and can be seen as an optical analog to the image-charge effect where a dipole-like image forms as schematically depicted in Fig. 3c . We note that in experiments further (blue or red) shifts might occur due to, e.g., strain or hybridization. Table 1 compares the bandgap, exciton and trion excitation, and binding energies for the analyzed substrates. As mentioned above, the red-shift of the A exciton is smaller than the red-shift of the A − trion. This results in a trion-binding energy \(E_{\mathrm{b}}^{{\mathrm{A}}^ - }\) that is substrate dependent. The corresponding values are also listed for the B − trion showing the same characteristics. On the Au(111) substrate \(E_{\mathrm{b}}^{{\mathrm{A}}^ - }\) gets reduced by more than 50%. The binding results from the Coulomb interactions between the hole and the two excited electrons. Weakening this interaction through screening thus leads to a weaker bond between the three particles. For the A − trion on SiO 2 , we find \(E_{\mathrm{b}}^{{\mathrm{A}}^ - } = 35\) meV, while the corresponding binding energy of the positive trion is slightly smaller with 32 meV. These values agree very well with experimental results with values between 20–43 meV [12] , [13] , [58] , [59] (on SiO 2 substrates). On the other hand, we note that absolute transition energies slightly deviate as discussed earlier [60] . In the case of a WSe 2 monolayer, a reduction of the trion-binding energy by ~10% was found by Lippert et al. [52] increasing the screening from an SiO 2 to a sapphire substrate. Furthermore, we are able to predict a binding energy of the B − trion of 23 meV in vacuum and 18 meV on SiO 2 (for B + 23 and 17 meV). Experimentally the B −/+ trion has been observed by reflectance measurements by Yang et al. [24] in WSe 2 and MoSe 2 . The additional doping by substrates in two-dimensional semiconducting TMDCs frequently results in the formation of trions. Taking an MoS 2 monolayer as representative, these were addressed by our novel theoretical framework. We could reveal the diversity of trion states with both resonant and bound trions. We find one energetically low, optically active A + trion, while A − shows a fine splitting into three excitations with inter- and intra-valley character. Our results explain recent experimental findings that showed more than one trion excitation. At higher energy, also the B excitons are accompanied by red-shifted B +/− trions. In addition, we have discussed the influence of three widely used substrates (SiO 2 , h -BN, and Au(111)). The additional screening renormalizes both the electronic gap, the exciton, and trion-binding energies. For the three investigated substrates, we find that the effects on the exciton and trion excitation energies do not exactly cancel each other, such that a shift always to lower energy is left. The trion-binding energies for the A − (A + ) trion of ~43 meV (~39 meV) in vacuum are slightly reduced on an SiO 2 substrate to ~35 meV (~32 meV). Our quantitative results concerning the binding energies as well as the magnitude of the A exciton red-shifts are in good agreement with experimental observations. Our findings are especially relevant since most possible opto-electronic applications involve substrates, which makes a deeper qualitative and quantitative understanding of the changes induced by the drastically enhanced screening environment essential both for excitons and trions. Bethe–Salpeter equation for excitons For the excitonic absorption spectra in Fig. 1 we solve the Bethe–Salpeter equation (BSE), starting from a preceding GW calculation within MBPT [61] , [62] (see also Supplementary Notes 1 and 2 ). In the self-energy operator of the GW, we employ the simplified LDA + GdW approximation [46] for numerical efficiency. Here, the dielectric screening properties are described by an atom-resolved model function based on the random-phase approximation [46] . The LDA + GdW approximation yields good results for the MoS 2 monolayer at a fraction of the numerical cost of a GW calculation, which is, e.g., used by Qiu et al. [60] who find the excitation energy of the A exciton as Ω A = 2.04 eV and Ω B = 2.17 eV. Our approach yields Ω A = 2.13 eV and Ω B = 2.29 eV. Equation of motion for trions The presented trion spectra and wave functions are obtained as eigenstates of an effective Hamiltonian (for negative trions) with matrix elements [40] 
    [                                         ⟨vc_1c_2| Ĥ^(eeh)|v'c_1'c_2'⟩                                                                -8pt = -7pt( ϵ _c_1 + ϵ _c_2 - ϵ _v)δ _c_1,c_1'δ _c_2,c_2'δ _v,v'    ( Ĥ_BS);                                                                                                                                                        + ( W_c_1c_2,c_1'c_2' - W_c_1c_2,c_2'c_1')δ _v,v'  ( Ĥ_ee);                                                                                                                                                      - ( W_v' c_1,vc_1' - V_v' c_1,c_1'v)δ _c_2,c_2'    ( Ĥ_eh,1);                                                                                                                                                      - ( W_v' c_2,vc_2' - V_v' c_2,c_2'v)δ _c_1,c_1'    ( Ĥ_eh,2) ]
 (1) (see also Supplementary Note 3 ). Here the short-hand notation v = ( v , k v ) is used for band index and k -vector. \(\epsilon _{{\bf{c}}_1}\) etc. denote the quasiparticle band-structure energies, V i the bare, and W i the screened Coulomb interaction \(W\left( {{\bf{r}},{\bf{r{\prime}}}} \right) = {\int} \varepsilon ^{ - 1}\left( {{\bf{r}},{\bf{r{\prime\prime}}}} \right)V\left( {{\bf{r{\prime\prime}}},{\bf{r{\prime}}}} \right)\mathrm{d}^3{\bf{r{\prime\prime}}}\) , where the dielectric function enters. The Hamilton matrix is constructed from four parts: the band structure term \(\hat H_{{\mathrm{BS}}}\) , electron–electron repulsion \(\hat H_{{\mathrm{ee}}}\) , and the attraction between the hole and both electrons \(\hat H_{{\mathrm{eh}},1/2}\) . Each of the last three is split into a direct part and an exchange part of the Coulomb interaction. The total momentum of the trion state is fixed and determines k 1 + k 2 − k v = K . Since the absorbed photon has nearly zero momentum, the total momentum of the trion is given by the momentum of the electron from which the trion state is excited. In the present study, this additional electron can reside in either one of the two lowest conduction bands (split by 15 meV) at the K points of the Brillouin zone (for the K = K transition the optical dipoles are found to be by far the strongest). Leaving out the second electron reduces Eq. ( 1 ) to the BSE Hamiltonian \(\left\langle {{\bf{vc}}\left| {\hat H^{({\mathrm{eh}})}} \right|{\bf{v{\prime}c{\prime}}}} \right\rangle = \left( {\epsilon _{\bf{c}} - \epsilon _{\bf{v}}} \right)\delta _{{\bf{cc{\prime}}}}\delta _{{\bf{vv{\prime}}}} - \left( {W_{{\bf{v{\prime}c}},{\bf{vc{\prime}}}} - V_{{\bf{v{\prime}c}},{\bf{c{\prime}v}}}} \right)\) , commonly used for excitons within MBPT [26] , [27] . The diagonalization of the trion Hamilton matrix is numerically extremely demanding due to the immense dimension of ~10 7 for a typical calculation and relies on recursive diagonalization schemes [63] , [64] . We apply a 27 × 27 × 1 k -space grid in the 2D Brillouin zone and include two valence and four conduction bands. Note that within our approach the A and B excitons and trions converge extremely fast with respect to the k -mesh. This is discussed in detail in Supplementary Figs. 3 – 6 . For all calculations presented in this work, a supercell of 45 Å perpendicular to the monolayer is used. Further numerical details of our calculations are discussed in Supplementary Notes 4 – 6 and Supplementary Figs. 1 and 2 . A detailed introduction to the method and the Hamilton matrix can be found in ref. [40] . We note that we do not include changes of the initial band structure due to additional carriers [65] , i.e., the presented spectra describe the limit of very-low doping. Positive trions can be described by the reformulation of Eq. ( 1 ) in which one of the excited electrons is replaced by an excited hole. Data availability The data that support the findings of this study are available from the corresponding author upon reasonable request.